Basal foot MTOC organizes pillar MTs required for coordination of beating cilia Coordination of ciliary beating is essential to ensure mucus clearance in the airway tract. The orientation and synchronization of ciliary motion responds in part to the organization of the underlying cytoskeletal networks. Using electron tomography on mouse trachea, we show that basal bodies are collectively hooked at the cortex by a regular microtubule array composed of 4–5 microtubules. Removal of galectin-3, one of basal-body components, provokes misrecruitment of γ-tubulin, disorganization of this microtubule framework emanating from the basal-foot cap, together with loss of basal-body alignment and cilium orientation, defects in cilium organization and reduced fluid flow in the tracheal lumen. We conclude that galectin-3 plays a crucial role in the maintenance of the microtubule-organizing centre of the cilium and the ‘pillar’ microtubules, and that this network is instrumental for the coordinated orientation and stabilization of motile cilia. In mammals, the epithelia lining the respiratory tracks, the oviduct and the brain ventricles contain multiple motile cilia that are numerous on the surface of differentiated epithelial cells. Defects in motile cilia lead to impaired fluid flow and generate respiratory disorders or infertility [1] , [2] , [3] . Motile cilia exhibit a 9+2-axonemal microtubule (MT) organization, and ciliary beating per se is attributed to the central microtubule doublets and the dynein arms present in the core of the axonemes. The coordination of cilium motion is controlled by the polarized organization of cilium bases at the apical domain of epithelial cells, as illustrated by basal feet aligned in the same direction. A number of mechanisms have been proposed to dictate basal-body (BB) cortical distribution [4] , [5] , [6] . In one of the proposed mechanisms, the distribution of planar cell polarity proteins influences the arrangement of BBs at the apical cortex [4] . For instance, in Xenopus embryos, the Dishevelled-2 mutation leads to impaired BB alignment [7] . Defective BB arrangement is also observed in mouse Vangl1 -mutant trachea [8] . In another proposed mechanism, fluid flow applied to ciliated cells is suggested to refine BB alignment in Xenopus embryos and in mouse ependymal cells, suggesting that there is a feedback loop of regulation [9] , [10] . In addition, the organization of the cortical cytoskeleton located in the apical domain of ciliated cells has been proposed as a factor that helps to establish polarization of BBs [11] , [12] . Galectin-3 is a member of the galectin family, a family of small soluble proteins that are conserved from invertebrates to vertebrates. These proteins have well-established roles in the progression of epithelial cancer and general immune response [13] . They have also been implicated in embryogenesis [14] and in various specific disorders, notably in the aggravation of polycystic kidney disease [15] , [16] . Galectin-3 is located at the primary cilia in renal epithelial cells [16] , [17] , [18] , and detailed examination of galectin-3-null mutant ( gal3−/− ) kidneys in adult mice revealed aberrant primary cilia, suggesting profound defects in ciliogenesis [18] . Interestingly, a recent report indicated that motile cilia of the ependymal cells were also affected in gal3−/− mice [19] . In addition, it is well known that gal3−/− mice are more sensitive to allergens and bacterial infections of their airways [20] , [21] , [22] , [23] . Therefore, studying the function of galectin-3 on the tracheal airway should highlight the role of this small molecule on ciliogenesis. Here, we demonstrate for the first time that galectin-3 is a basal-foot cap component. Loss of galectin-3 leads to impaired recruitment of γ-tubulin at that level. We show that the MT network emanating from the BBs is disrupted, leading to perturbed ciliary organization and fluid movement in mutant mouse airways. Defective organization of motile cilia in gal3−/− tracheas We analysed motile cilium morphology in the tracheal epithelium of wild-type (wt) and gal3−/− adult mice using scanning electron microscopy (SEM) ( Fig. 1 ). In this tissue, multiciliated cells are interspersed with smooth secreting cells. Low-magnification views revealed entanglements of irregular cilia and large swellings of the membrane at the epithelial surface of gal3−/− biopsies when compared with the regular arrangement of wt epithelium ( Fig. 1a,b ). At higher magnifications, it is clear that individual gal3−/− cells have cilia that are often flattened, tapered and seem to be heterogeneous in length, shape, diameter and orientation when compared with wt cells ( Fig. 1c,d ). However, gal3−/− ciliary sets display only a slight length increase in comparison with wt ones ( Supplementary Fig. 1A and B ). No obvious defect has been observed in the distribution of intraflagellar transport (IFT) proteins such as IFT88 ( Supplementary Fig. 1C ). Moreover, transmission electron microscopy (TEM) analyses showed that transversal views of the gal3−/− axonemes displayed more defects in the classical 9+2-MT organization of motile cilia, such as incomplete or even sometimes absent MT central pairs, or incomplete or displaced outer MT pairs, than in wt axonemes ( Fig. 1e–k ). We conclude that the absence of galectin-3 perturbs the correct organization of mouse tracheal motile cilia. 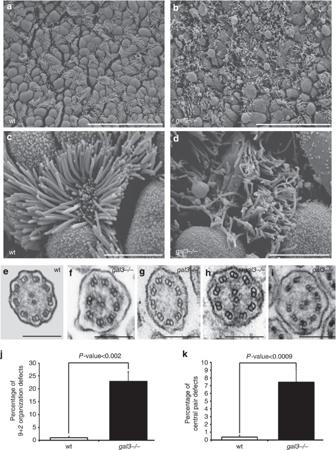Figure 1: Defective motile cilium organization in mousegal3−/−tracheas. (a–d) The luminal surface of wt (a,c)(N=4 wt mice) andgal3−/−(b,d)(N=4gal3−/−mice) tracheal epithelium was analysed using SEM. Low magnifications (a,b) and high magnifications (c,d) are presented. Scale bars, 20 μm (a,b) and 5 μm (c,d). (e–i) TEM ultrastructural analyses of axonemal transverse sections in wt (e) andgal3−/−(f–i) tracheas. Scale bar, 200 nm (e–i). (j) Statistical analysis of the 9+2-axonemal organization defects in wt (white) andgal3−/−(black) tracheas. Mann–Whitney test,P-value=0.0019.N(wt)=9 mice,n(wt)=305 cilia;N(gal3−/−)=9 mice,n(gal3−/−)=940 cilia. (k) Statistical analysis of the central-pair defects in wt (white) andgal3−/−(black) tracheas. Mann–Whitney test,P-value=0.00087.N(wt)=9 mice,n(wt)=889 cilia;N(gal3−/−)=9 mice,n(gal3−/−)=599 cilia. Values are mean±s.e.m. Figure 1: Defective motile cilium organization in mouse gal3−/− tracheas. ( a – d ) The luminal surface of wt ( a , c ) (N =4 wt mice) and gal3−/− ( b , d ) (N =4 gal3−/− mice) tracheal epithelium was analysed using SEM. Low magnifications ( a , b ) and high magnifications ( c , d ) are presented. Scale bars, 20 μm ( a , b ) and 5 μm ( c , d ). ( e – i ) TEM ultrastructural analyses of axonemal transverse sections in wt ( e ) and gal3−/− ( f – i ) tracheas. Scale bar, 200 nm ( e – i ). ( j ) Statistical analysis of the 9+2-axonemal organization defects in wt (white) and gal3−/− (black) tracheas. Mann–Whitney test, P -value=0.0019. N (wt)=9 mice, n (wt)=305 cilia; N ( gal3−/− )=9 mice, n ( gal3−/− )=940 cilia. ( k ) Statistical analysis of the central-pair defects in wt (white) and gal3−/− (black) tracheas. Mann–Whitney test, P -value=0.00087. N (wt)=9 mice, n (wt)=889 cilia; N ( gal3−/− )=9 mice, n ( gal3−/− )=599 cilia. Values are mean±s.e.m. Full size image Defective rotational polarity in gal3−/− tracheas To further analyse the cortical organization of motile cilia within individual cells, we measured the relative orientation of central MT doublets and basal feet in ciliary sets on wt and gal3−/− tracheal samples by TEM ( Fig. 2 ). The mean angular deviation of the central MT doublets from neighbouring cilia was 23.01° in wt cells compared with 39.19° in gal3−/− cells ( Fig. 2a–c ). There was an even larger effect on the mean circular deviation of the basal feet within individual cells (mean r cell ( gal3−/− )=0.737±0.027 versus mean r cell (wt)=0.978±0.003) ( Fig. 2d–f ). Cortical displacement or clustering of BBs was never observed in gal3−/− tracheas ( Fig. 2d,e ). We measured BB directionality at the tissue level in mutant mice. The intercellular coordination of BB orientation across the trachea was mildly perturbed in gal3−/− tracheas ( r trachea ( gal3−/− )=0.729 versus r trachea (wt)=0.976). Together, these results demonstrate that galectin-3 is essential for the proper orientation of BBs and subsequently of the axonemes. 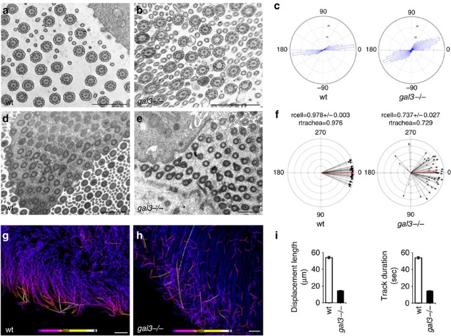Figure 2: Cilium organization and flow directionality are lost in mousegal3−/−ciliated cells. TEM ultrastructural analysis of axonemal (a,b) and BB (d,e) transversal sections in wt andgal3−/−mouse tracheas. Scale bars, 1 μm (a,b,dande). (c) Statistical analyses of central MT-pair orientation in individual cells with MATLAB. wt cilium mean angular deviation: ±23.01°;gal3−/−cilium mean angular deviation: ±39.19°; Watson–Wheeler homogeneity test,P-value=6.91 × 10−15.N(wt)=8 mice,n(wt)=338 axonemes;N(gal3−/−)=7 mice,n(gal3−/−)=411 axonemes. (f) Statistical analyses of BB orientation in individual cells and along the tracheal axis with Oriana2.0.rcell(wt)=0.978±0.003;rtrachea(wt)=0.976;rcell(gal3−/−)=0.737±0.027;rtrachea(gal3−/−)=0.729.N(wt)=3 mice,n(wt)=284 basal feet;N(gal3−/−)=3 mice,n(gal3−/−)=341 basal feet. (g,h) Representative patterns of fluorescent bead dynamics above wt (g) andgal3−/−(h) tracheal explants. Scale bar, 30 μm. (i) Statistical analyses of fluorescent bead behaviour on the surface of wt (white) andgal3−/−(black) tracheal epithelia. Fluorescent bead track displacement lengths and durations were automatically measured using Imaris software.N(wt)=6 mice, one tracheal ring per animal,n(wt)=3,981 tracked beads;N(gal3−/−)=6 mice, 1 tracheal ring per animal,n(gal3−/−)=11,156 tracked beads.N(wt track displacement length)=49±0.8 μm,n(wt track duration)=53.84±1.34 s,n(gal3−/−track displacement length)=29.63±0.29 μm,n(gal3−/−track duration)=14.57±0.22 s. Values are mean±s.e.m. Figure 2: Cilium organization and flow directionality are lost in mouse gal3−/− ciliated cells. TEM ultrastructural analysis of axonemal ( a , b ) and BB ( d , e ) transversal sections in wt and gal3−/− mouse tracheas. Scale bars, 1 μm ( a , b , d and e ). ( c ) Statistical analyses of central MT-pair orientation in individual cells with MATLAB. wt cilium mean angular deviation: ±23.01°; gal3−/− cilium mean angular deviation: ±39.19°; Watson–Wheeler homogeneity test, P -value=6.91 × 10 −15 . N (wt)=8 mice, n (wt)=338 axonemes; N ( gal3−/− )=7 mice, n ( gal3−/− )=411 axonemes. ( f ) Statistical analyses of BB orientation in individual cells and along the tracheal axis with Oriana2.0. r cell (wt)=0.978±0.003; r trachea (wt)=0.976; r cell ( gal3−/− )=0.737±0.027; r trachea ( gal3−/− )=0.729. N (wt)=3 mice, n (wt)=284 basal feet; N ( gal3−/− )=3 mice, n ( gal3−/− )=341 basal feet. ( g , h ) Representative patterns of fluorescent bead dynamics above wt ( g ) and gal3−/− ( h ) tracheal explants. Scale bar, 30 μm. ( i ) Statistical analyses of fluorescent bead behaviour on the surface of wt (white) and gal3−/− (black) tracheal epithelia. Fluorescent bead track displacement lengths and durations were automatically measured using Imaris software. N (wt)=6 mice, one tracheal ring per animal, n (wt)=3,981 tracked beads; N ( gal3−/− )=6 mice, 1 tracheal ring per animal, n ( gal3−/− )=11,156 tracked beads. N (wt track displacement length)=49±0.8 μm, n (wt track duration)=53.84±1.34 s, n ( gal3−/− track displacement length)=29.63±0.29 μm, n ( gal3−/− track duration)=14.57±0.22 s. Values are mean±s.e.m. Full size image Since interconnection between cilium organization and coordinated motion has been reported [7] , we next prepared tracheal explants to test the consequences of galectin-3 depletion on ciliary functions. Several randomly ciliated cells from each of the tracheal samples were finely imaged using high-resolution camera recordings. In Supplementary Movie 1 , wt ciliary sets generate a coordinated and regular wave-like movement, as previously described [24] , [25] . In contrast, the gal3−/− collective beating profile appeared asynchronous ( Supplementary Movie 2 ). Ciliary movements were barely detectable in our hands on very few mutant tracheas. In addition, the flow generated by ciliary beating was studied by monitoring particle transport above the mouse tracheal epithelia. Movements of fluorescent beads were followed above the epithelial cell monolayer on tracheal explants from wt and gal3−/− mice by live imaging ( Supplementary Movies 3 and 4 ). The entire fluorescent bead populations were automatically tracked. Bead-tracking landscapes revealed that the direction of the flow was uncoordinated in gal3−/− explants when compared with wt explants ( Fig. 2g,h ). We noticed that the displacement length and duration of the bead movements were reduced in mutant mice compared with wt mice ( Fig. 2i ), demonstrating a strong decrease in the efficiency of particle transport in the absence of galectin-3. Taken together, these data show that galectin-3 is required for an efficient synchronous and coordinated ciliary beating pattern and for efficient fluid flow on the surface of ciliated cells. This is important as in vivo ciliated cells located on the airway epithelium normally ensure the direct transport of mucus. Given the abnormalities we observed, we examined tracheal mucus displacement in mutant mice. Using SEM analyses, we noticed the frequent accumulation of thin mucus layers over the tracheal epithelium of mutant mice ( Supplementary Fig. 2A and B ), which was confirmed by Alcian blue staining of mucus on paraffin sections ( Supplementary Fig. 2C and D ). Therefore, the inefficient flow generated at the surface of ciliated cells is associated with defects in tracheal mucus clearance in gal3−/− mice. Altogether, these results demonstrate that coordinated ciliary motility is defective in the absence of galectin-3. Galectin-3 is associated with the MTOC at the cilium base How can galectin-3 affect the organization of motile cilia? We first analysed the distribution of endogenous galectin-3 in tracheal ciliated cells of adult mice. Immunostaining and confocal analyses revealed that galectin-3 is present throughout the cytoplasm, with a strong enrichment at the apical cortex ( Fig. 3a,b ). Double immunostainings with acetylated α-tubulin showed that galectin-3 is located at the base of the motile cilium ( Fig. 3a,b ). To visualize galectin-3 localization, we next performed immunogold staining on ultrathin sections of wt tracheas, using ultrathin sections of gal3−/− tracheas as negative controls. Galectin-3 was detected at the ciliary rootlet and at the basal-foot cap ( Fig. 3c , black arrows and black arrowheads, respectively). Basal-foot caps and ciliary rootlets have been suggested to be the MT-anchoring sites of the BB, and are now considered as the MT-organizing centres (MTOCs) of the cilium base [26] , [27] , [28] . Consistently, immunogold staining revealed that γ-tubulin is located at the basal-foot cap and at the ciliary rootlet in mouse tracheal multiciliated cells ( Fig. 3d , arrows and arrowheads, respectively), as previously observed in oviduct epithelial cells [27] . Given galectin-3 localization with the basal-foot cap, we conclude that this lectin is associated with the cilium base MTOC. Interestingly, the number of γ-tubulin gold particles is significantly decreased at the basal-foot cap in mutant tracheas ( Fig. 3e ), showing that γ-tubulin is misrecruited at the cilium base MTOC in the absence of galectin-3. 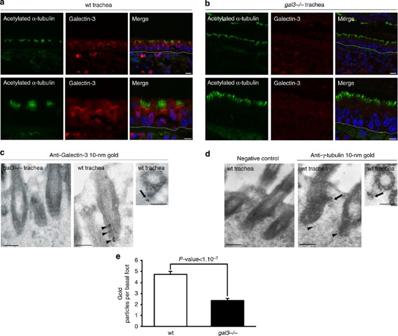Figure 3: Galectin-3 is present at the basal-foot cap and ciliary rootlet of motile cilium in tracheal epithelial cells. (a) Confocal microscopy analysis of galectin-3 distribution in mouse tracheal cells. Longitudinal paraffin sections were immunostained with monoclonal anti-acetylated α-tubulin (green) and polyclonal anti-galectin-3 (red) antibodies. (b)Gal3−/−mouse tracheas were used as a negative control for galectin-3 immunofluorescence. Galectin-3 is highly enriched at the cilium base of tracheal epithelial cells. Nuclei were detected by Hoechst 33342 staining (blue). Tracheal epithelium is demarcated by a white dotted line. Scale bars, upper panel 10 μm, lower panel 5 μm. (c,d) TEM ultrastrural analyses of galectin-3 (c) and γ-tubulin (d) localizations at the BBs. Lowicryl sections were immunostained with monoclonal anti-galectin-3 or polyclonal anti-γ-tubulin antibodies.Gal3−/−mouse tracheas were used as a negative control for galectin-3 immunogold staining (c). Incubation of the sections with only the secondary antibody was used as a negative control (d). Scale bar, 300 nm. (e) Statistical analysis of the number of γ-tubulin gold particles per basal foot in wt (white) andgal3−/−(black). Mann–Whitney test,P-value=1.283 × 10−8.N(wt)=3 mice,n(wt)=67 basal feet;N(gal3−/−)=3 mice,n(gal3−/−)=50 basal feet. Values are mean±s.e.m. Figure 3: Galectin-3 is present at the basal-foot cap and ciliary rootlet of motile cilium in tracheal epithelial cells. ( a ) Confocal microscopy analysis of galectin-3 distribution in mouse tracheal cells. Longitudinal paraffin sections were immunostained with monoclonal anti-acetylated α-tubulin (green) and polyclonal anti-galectin-3 (red) antibodies. ( b ) Gal3−/− mouse tracheas were used as a negative control for galectin-3 immunofluorescence. Galectin-3 is highly enriched at the cilium base of tracheal epithelial cells. Nuclei were detected by Hoechst 33342 staining (blue). Tracheal epithelium is demarcated by a white dotted line. Scale bars, upper panel 10 μm, lower panel 5 μm. ( c , d ) TEM ultrastrural analyses of galectin-3 ( c ) and γ-tubulin ( d ) localizations at the BBs. Lowicryl sections were immunostained with monoclonal anti-galectin-3 or polyclonal anti-γ-tubulin antibodies. Gal3−/− mouse tracheas were used as a negative control for galectin-3 immunogold staining ( c ). Incubation of the sections with only the secondary antibody was used as a negative control ( d ). Scale bar, 300 nm. ( e ) Statistical analysis of the number of γ-tubulin gold particles per basal foot in wt (white) and gal3−/− (black). Mann–Whitney test, P -value=1.283 × 10 −8 . N (wt)=3 mice, n (wt)=67 basal feet; N ( gal3−/− )=3 mice, n ( gal3−/− )=50 basal feet. Values are mean±s.e.m. Full size image BB-associated MT network is altered in gal3−/− tracheas To examine the detailed organization of the MT network at the base of the cilium and the consequences of galectin-3 depletion, we used dual-axis electron tomography on the apical cortical domain of ciliated cells and acquired tomograms from wt and gal3−/− mouse trachea samples (see representative tomogram stacks of wt and gal3−/− tracheas in Supplementary Movies 5 and 7 , and Supplementary Movies 6 and 8 , respectively). Reconstructions of the wt tracheas showed arrays of MTs emanating from the basal foot ( Fig. 4a,c ). A few MTs run parallel to the apical surface and connect neighbouring ciliary rootlets, but the majority is orientated obliquely and perpendicularly to the surface and point towards the cell centre. This network is composed of 4–5 MTs emanating from each basal-foot cap ( Fig. 4a,c and g ). Interestingly, no interaction between basal-foot caps or ciliary rootlets and actin microfilaments was observed. In fact, the actin cytoskeleton was barely detectable on tomographic sideviews of this cortical region, but was readily seen in tomographic top views as sinuous interwoven microfilaments between BBs ( Supplementary Fig. 3 , Supplementary Movies 7 and 8 , Fig. 5 ). In gal3−/− tracheas, only a few MTs were detected in this region, with an average of 1.5 microtubules connected to the basal-foot cap ( Fig. 4b,d and g ). Abnormal accumulation of intracellular organelles such as endoplasmic reticulum tubules and mitochondria were also visible in gal3−/− tracheas, possibly reflecting the absence of MT-derived steric hindrance in this part of the cytoplasm ( Fig. 4b,d ). The absence of galectin-3 did not have any detectable effect on the actin meshwork in this region ( Supplementary Fig. 3 , Supplementary Movies 7 and 8 , Fig. 5 ). Models generated from EM tomograms clearly showed that the association of MTs with BBs is strongly reduced in gal3−/− tracheas in comparison with wt tracheas ( Fig. 4e,f ). We conclude that galectin-3 is required to organize the MT framework with BBs in mouse tracheas ( Fig. 5 ). 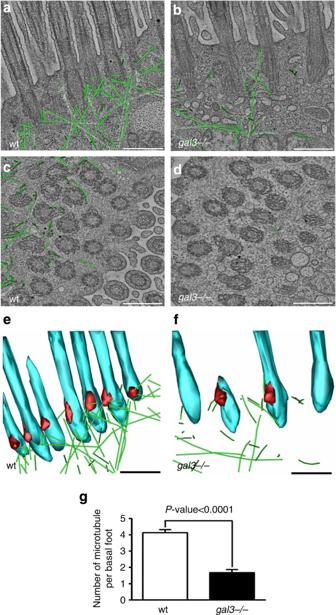Figure 4: Association of MTs with basal feet is severely disrupted ingal3−/−mouse tracheas. Representative EM tomographic slices, generated by averaging fivez-sections of the reconstructed filtered volume, of the cortical domain of wt (a,c) andgal3−/−(b,d). Ciliated cells are presented with superimposition of the contour of the MTs (green). The identification of a MT is based on its shape and diameter (20 nm). Longitudinal (a,b) and transversal (c,d) sections are shown. (e,f) Three-dimensional (3D) models of the EM tomographic reconstructions of cilium base (blue), basal foot (red) and MTs (green) were generated for wt (e) andgal3−/−(f) ciliated cells, and representative tilted longitudinal views are presented. Scale bar, 500 nm. (g) Statistical analysis of the number of MTs per basal foot in wt (white) andgal3−/−(black). Mann–Whitney test,P-value=3.18 × 10−12.N(wt)=3 mice,n(wt)=60 basal feet;N(gal3−/−)=3 mice,n(gal3−/−)=53 basal feet. Values are mean±s.e.m. Figure 4: Association of MTs with basal feet is severely disrupted in gal3−/− mouse tracheas. Representative EM tomographic slices, generated by averaging five z -sections of the reconstructed filtered volume, of the cortical domain of wt ( a , c ) and gal3−/− ( b , d ). Ciliated cells are presented with superimposition of the contour of the MTs (green). The identification of a MT is based on its shape and diameter (20 nm). Longitudinal ( a , b ) and transversal ( c , d ) sections are shown. ( e , f ) Three-dimensional (3D) models of the EM tomographic reconstructions of cilium base (blue), basal foot (red) and MTs (green) were generated for wt ( e ) and gal3−/− ( f ) ciliated cells, and representative tilted longitudinal views are presented. Scale bar, 500 nm. ( g ) Statistical analysis of the number of MTs per basal foot in wt (white) and gal3−/− (black). Mann–Whitney test, P -value=3.18 × 10 −12 . N (wt)=3 mice, n (wt)=60 basal feet; N ( gal3−/− )=3 mice, n ( gal3−/− )=53 basal feet. Values are mean±s.e.m. 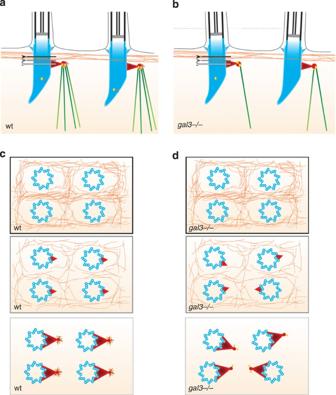Figure 5: Schemes showing the predicted association of the MT network and the actin cytoskeleton with the basal bodies of motile cilia from the acquired tomograms. Side (a,b) or top (c,d) views are presented for wt (a,c) andgal3−/−(b,d) ciliated cells. MTs (green), actin cables (orange), galectin-3 (purple) and γ-tubulin (yellow) are represented at the BBs (blue) and at the basal-foot cap (red). The relative position of the actin cytoskeleton to the basal foot in wt (a) andgal3−/−(b) is showed with black (above the basal foot), grey (the top of the basal foot) and white (at the level of the basal-foot cap) arrows and lines. (c,d) Black, grey and white panels correspond to black, grey and white line positions inaandb. Full size image Figure 5: Schemes showing the predicted association of the MT network and the actin cytoskeleton with the basal bodies of motile cilia from the acquired tomograms. Side ( a , b ) or top ( c , d ) views are presented for wt ( a , c ) and gal3−/− ( b , d ) ciliated cells. MTs (green), actin cables (orange), galectin-3 (purple) and γ-tubulin (yellow) are represented at the BBs (blue) and at the basal-foot cap (red). The relative position of the actin cytoskeleton to the basal foot in wt ( a ) and gal3−/− ( b ) is showed with black (above the basal foot), grey (the top of the basal foot) and white (at the level of the basal-foot cap) arrows and lines. ( c , d ) Black, grey and white panels correspond to black, grey and white line positions in a and b . Full size image In this study, we identified galectin-3 at the base of the motile cilia in tracheal cells, confirming and extending the original reports showing galectin-3 at the base of the primary cilium in renal cells [16] , [17] , [18] . Immunogold experiments revealed that galectin-3 is located at the BB, more specifically at the basal-foot caps and the ciliary rootlets in multiciliated tracheal cells. To date, only γ-tubulin and ODF2 have been localized to basal-foot caps [27] , [28] . We show that galectin-3 is also localized at the basal-foot cap, indicating that it is associated with the (−) end of MTs at nucleation/anchoring sites at the BB. In gal3−/− trachea, the absence of galectin-3 had a drastic effect on the MT network, and the cytoplasmic MT array was extremely sparse in the cortical domain. These data strongly suggest that galectin-3 might be associated with the motile cilium MTOC, where it participates in MT nucleation and/or stabilization, and are in agreement with previous studies reporting that there is a transient association of galectin-3 with the centrosome, the main MTOC in interphase epithelial cells [16] , [18] . Perturbation of the subciliary MT network at the base of the cilium had direct consequences on BB organization. The BBs were normally spaced but their alignment was impaired in gal3−/− multiciliated cells, clearly showing that rotational cell polarity is disrupted in the absence of galectin-3. It has long been observed that the cytoskeletal network interacts with BBs [29] , but more recent data suggest that the polarized arrangement of BBs depends on the sequential involvement of actin and microtubules. First, the docking of BBs at the plasma membrane and their relative spacing at the apical cortex appear to be driven by the actin cytoskeleton [11] , [30] ; next, the cortical MT network seems to be important for the rotational polarity of BBs. This conclusion is based on the results of nocodazole treatments on frog or mouse multiciliated cells [8] , [11] and on the study of Odf2-mutant mice lacking the entire basal-foot structures [28] . However, direct evidence is still missing and the exact mechanism remains unclear. Here, removing a protein associated with the basal feet using a genetic approach was sufficient to perturb the recruitment of γ-tubulin at the basal-foot cap, and to severely affect cortical MTs and subsequently BB alignement. Together, these results pinpoint the importance of these protein complexes at the level of the basal-foot cap and further emphasize the long-standing hypothesis that this BB appendage is a cilium MTOC [26] , [27] . Since the MT network has been reported to participate in planar cell polarity establishment and signalling [5] , [8] , [11] , it will be interesting to analyse the consequences of BB-associated MT perturbation on the distribution of planar cell polarity components. Analysing the structure of the cortical cytoskeleton using electron tomography, we show that MT and actin networks are independently organized in tracheal cells. On one hand, we observed sinuous actin microfilaments forming a dense meshwork encircling the BBs ( Fig. 5a,c and Supplementary Movie 7 ) and this organization is unchanged in galectin-3-mutant mice ( Fig. 5b,d and Supplementary Movie 8 ). This result is compatible with a previously assigned role in BB spatial distribution at the apical surface. On the other hand, the cortical cytoplasmic MTs originate from the BBs, mainly from the basal-foot caps. Most of the MTs are orientated obliquely and perpendicularly, with only a few that run parallel to the apical membrane connecting neighbouring BBs. The dual-axis electron tomography procedure we used allows higher image resolution [31] , [32] and reveals a different cytoskeletal organization at the BBs than the one proposed by Kunimoto et al . [28] Our data extend previous results obtained by TEM or immunofluorescence analyses [11] , [26] . Here we show that cilia do exist in gal3 −/− tracheas, but their structure, organization and function are affected. The axonemal abnormalities we observed could be the result of unstabilized BBs in the cortical domain of mutant ciliated cells. Indeed, it has been recently reported that ciliogenesis also depends on the stability of BBs in Tetrahymena [33] , [34] . Another possibility could be that BB-associated MTs behave as tracks to ensure the transport of soluble proteins at the ciliary base and thus to maintain a correct cilium structure (for review, see ref. 35 ). Reduction of MTs at the BBs may impair ciliary protein trafficking and thus ciliary access. Further experiments will be required in the future to test these hypotheses. In addition, we show that the loss of the BB-associated MTs is concomitant with impaired BB directionality and uncoordinated sets of motile cilia. The cortical MT network has been proposed to participate in BB positioning, and there could be a direct causal link between MTOC perturbation and BB misalignment in gal3−/− tracheas. Axonemal abnormalities and BB misalignment may then both explain ciliary beating deficiency and the inefficient flow production in the tracheal lumen of mutant mice. However, even if the axonemal abnormalities are present in weak proportion in mutant tracheas ( Fig. 1 ), we cannot exclude the possibility that they could alone be responsible for the generation of the inappropriate tracheal flow. It has been demonstrated that fluid flow per se exerts a feedback loop regulation of BB distribution [9] , [10] . Thus BB misalignment could also be a consequence of the defective fluid flow in gal3−/− tracheas. In summary, our data reinforce the concept that the basal-foot cap is the main cilium base MTOC. In fully differentiated tissues, we show that the subciliary MT array consists of regular and constant assemblies of 4–5 MTs per MTOC ( Figs 4 and 5 ). The cortical MTs may behave as cilium ‘pillars’. It is tempting to hypothesize that this MT framework, together with protein complexes located at the basal-foot cap, are a structural and functional unit of the motile cilium. Collectively, these units may form a retaining structure providing the mechanical resistance required to not only polarize and stabilize BBs, but also to maintain the overall cilium structure at the plasma membrane and withstand forces generated by cilium beating. Reagents and antibodies Rat (dilution 1:50) and rabbit polyclonal (1:100) antibodies directed against galectin-3 were kindly provided by Dr H. Leffler (Lund University, Sweden) and Dr H.P. Elsässer (Philipps University, Marburg), respectively. Monoclonal anti-acetylated α-tubulin (clone 6-11B-1, 1:200) and γ-tubulin (clone GTU-88, 1:50) were from Sigma (Saint-Louis, MO) and Abcam (Cambridge), respectively. Rabbit polyclonal IFT88 (1:100) was from Proteintech (Chicago, IL). Anti-mouse Alexa-488 and anti-rabbit Alexa-568 secondary antibodies (1:250) were from Life Technologies (Paisley, UK). Animals Wt and galectin-3-null mutant ( gal3−/−) [36] mice used here were of the 129Sv background. The animals were maintained in a specific pathogen-free animal house facility, and handled in accordance with the French regulation for animal care. A total of N =43 wt and N =43 gal3−/− male adult mice were used. All samples were number coded for blind experiments. Three-month-old mice were killed by cervical dislocation. After the thorax was opened, the submandibular gland and the infrahyoid musculature were removed. The trachea was cut at the borders between the larynx and the bronchial bifurcation, and processed as follows. Immunohistochemistry and immunofluorescence microscopy Two fixation procedures were used. Samples were incubated overnight at 4 °C in Carnoy fixative (60% ethanol, 30% chloroform, 10% acetic acid) and stored in 70% ethanol. Alternatively, samples were fixed overnight at 4 °C in 70% methanol, followed by 1 day at 4 °C in 100% methanol, and then stored at −20 °C in methanol. N =8 wt and N =8 gal3−/− tracheas were paraffin-embedded for sectioning. Sections (5 μm) were de-waxed in a xylene bath, rehydrated once in isopropanol, then in decreasing ethanol solutions, and were processed for either immunohistochemistry or immunostaining. Mucus was detected by Alcian blue staining, and nuclei were then detected by Nuclear Fast Red incubation. Images were acquired using an Eclipse 90i Upright microscope and a coolSNAP HQ2 CCD colour camera (Nikon, Tokyo). For immunostaining, de-waxed tissue sections were blocked in 1.5% donkey serum (Sigma) for 1 h. Primary antibody incubations were performed at 4 °C for 12 h, and secondary antibody incubations at room temperature for 2 h, both in 1.5% donkey serum solution. Hoechst 33342 staining (Life Sciences) was used to detect nuclei. Tissue sections were mounted in Mowiol488 solution. Confocal images of fixed cells were acquired on a Leica TCS SP5 microscope using a × 63 and a × 100 lens (Leica Microsystems, Wetzlar, Germany). Ex vivo analyses of tracheal epithelial cells Tracheal explants were prepared from N =7 wt and N =7 gal3−/− mice according to Delmotte and Sanderson [24] , with minor modifications. The trachea were removed and sliced into 0.5-mm-wide rings. The rings were washed three times in pre-warmed DMEM 4.5 g l −1 glucose medium (Life Technologies) complemented with 25 mM HEPES (pH 7.4) and mounted in a home-made chamber, in the same medium. This experiment was carried out using three tracheal explants per animal. Video acquisitions of cilium beating profile were performed using a LEICA DMI6000, a high-resolution camera CoolSnap HQ2 (Photometrics, Tucson, AZ) and MetaMorph 6 software (Molecular Devices, Sunnyvale, CA). It was performed on N =7 wt and N =7 gal3−/− mice, using three tracheal explants per animal. To record ciliary flow, suspensions of 0.2 μm fluorescent polystyrene beads (Sigma) were applied on N =6 wt and N =6 gal3−/− tracheal rings. Automatic bead tracking and movement calculations were performed using IMARIS 7.0 (Bitplane, Zurich). EM analyses For TEM analyses, tissue samples were isolated from N =8 wt and N =7 gal3−/− mouse tracheas, cut into small rings of about 1 mm and immersion-fixed overnight at 4 °C in 1.6% glutaraldehyde in Milloning buffer (0.1 M Na 2 HPO 4 , 0.1 M NaH 2 PO 4 , pH 7.3). Standard procedures for dehydration and embedding in Epon-Araldite (Electron Microscopy Sciences, Hatfield, PA) were used [37] . Semi-thin sections were stained with methylene blue and azur II. The ciliary length was measured on semi-thin sections of N =3 wt and N =3 gal3−/− mice, n (wt)=74 cells, n ( gal3−/− )=101 cells. Ultrathin sections were stained with uranyl acetate and lead citrate solutions before examination using a Tecnai T12 microscope (FEI, Eindhoven, The Netherlands). For SEM, N =4 wt and N =4 gal3−/− longitudinal trachea sections were immersion-fixed overnight at 4 °C in 1.6% glutaraldehyde in Milloning buffer. The samples were dehydrated by passing through a graded series of ethanol solutions, then dried by the CO 2 critical-point method and coated with a 20–40-nm gold thin layer using Scancoat Six (HHV, Crawley, UK). Acquisitions were performed using a Cambridge Stereoscan 260 (Cambridge Instruments, Somerville, MA). N =4 wt and N =4 gal3−/− tracheas were processed for immunogold experiments and TEM analyses. Tissue samples were fixed overnight in 1% formaldehyde, 0.1% glutaraldehyde, 0.1 M cacodylate buffer, pH 7.4 and then embedded in Lowicryl K4M resin (Polysciences, Warrington, PA). Ultrathin sections were treated with 1% bovine serum albumin before incubation in rat monoclonal anti-galectin-3 or in mouse monoclonal anti-γ-tubulin antibody, followed by 10-nm immunogold-conjugated goat anti-rat or anti-mouse antibody solution (British Biocell International, Cardiff, UK), respectively. Tomographic analyses Sections (300 nm) from mouse tracheal Epon blocks of N =3 wt and N =3 gal3−/− were cut using a Leica UC7 microtome (Leica Microsystems, Milton Keynes, UK). The sections were mounted on formvar-coated copper 133 mesh finder grids (Agar, Stansted, UK), which were subsequently coated on both sides with 10-nm protein-A gold (EMS, Hatfield, PA). Dual-axis tilt series were collected from −66° to +66° at 2° intervals with SerialEM [38] at a magnification of × 19,000 using a defocus of −0.5 μm on Tecnai F20 microscope (FEI) equipped with a Gatan 4k CCD camera (UltraScan 4000) (Gatan, Abingdon Oxon, UK). The tilt series were aligned and reconstructed using IMOD software [31] , [39] ( http://bio3d.colorado.edu/imod/ ). The reconstructions were then filtered using nonlinear anisotropic diffusion [40] implemented in IMOD. The segmentation of the tomograms shown in Fig. 4e and Supplementary Fig. 3 was performed manually in IMOD. Differences between microtubules and actin were based on fibre diameter. Measurement of axoneme and BB orientation Axoneme orientation was assessed by measuring central-pair orientation in individual cells on TEM acquisitions. Statistical analyses were performed with MATLAB software (MathWorks) and displayed in circular plots bidirectionally. N (wt)=8 mice, with n (wt)=338 axonemes and N ( gal3−/−) =7 mice with n ( gal3−/− )=411 axonemes. BB orientation was assessed as previously reported [9] . Tracheas were orientated according the lung–mouth axis during fixation. After TEM acquisitions, statistical analyses were performed using Oriana2.0 software (Kovach Computing Services, UK). Results are shown in circular plots in which each black vector represents the mean orientation of BBs in individual cells. Length of the black vector ( r cell ) is the complement of the circular variance and illustrates BB coordination. The red vector illustrates the intercellular coordination of orientation across the trachea and its length ( r t rachea ), the complement of the variance of individual cell mean orientation (black vector orientation). N (wt)=3 mice, n (wt)=40 cells and n (wt)=284 BBs; N ( gal3−/− )=3 mice, n ( gal3−/− )=52 cells and n ( gal3−/− )=343 BBs. How to cite this article: Clare, D. K. et al . Basal foot MTOC organizes pillar MTs required for coordination of beating cilia. Nat. Commun. 5:4888 doi: 10.1038/ncomms5888 (2014).